Ectopic expression of the histone methyltransferase Ezh2 in haematopoietic stem cells causes myeloproliferative disease Recent evidence shows increased and decreased expression of Ezh2 in cancer, suggesting a dual role as an oncogene or tumour suppressor. To investigate the mechanism by which Ezh2-mediated H3K27 methylation leads to cancer, we generated conditional Ezh2 knock-in (Ezh2-KI) mice. Here we show that induced Ezh2 haematopoietic expression increases the number and proliferation of repopulating haematopoietic stem cells. Ezh2-KI mice develop myeloproliferative disorder, featuring excessive myeloid expansion in bone marrow and spleen, leukocytosis and splenomegaly. Competitive and serial transplantations demonstrate progressive myeloid commitment of Ezh2-KI haematopoietic stem cells. Transplanted self-renewing haematopoietic stem cells from Ezh2-KI mice induce myeloproliferative disorder, suggesting that the Ezh2 gain-of-function arises in the haematopoietic stem cell pool, and not at later stages of myelopoiesis. At the molecular level, Ezh2 regulates haematopoietic stem cell-specific genes such as Evi-1 and Ntrk3, aberrantly found in haematologic malignancies. These results demonstrate a stem cell-specific Ezh2 oncogenic role in myeloid disorders, and suggest possible therapeutic applications in Ezh2-related haematological malignancies. Haematopoiesis is initiated by a small population of multipotent long-term haematopoietic stem cells (LT-HSCs) present in bone marrow that self-renew to maintain the quiescent HSC pool. On activation, LT-HSCs give rise to short-term HSCs (ST-HSCs), which further mature into the multipotent progenitors (MPP) that can differentiate to produce terminally differentiated haematopoietic cells [1] . Among the key epigenetic repressors required for the maintenance of transcriptional silencing in stem cells are the Polycomb group (PcG) proteins. PcG proteins are involved in regulating embryonic development, stem cell renewal and tumorigenesis [2] . PcG proteins exist as three multiprotein complexes: Polycomb repressive complexes (PRC) 1 and 2, and pleiohomeotic repressive complex [3] . PRC1 monoubiquitylates Lys 119 of histone H2A (H2AK119Ub) via RING1A and RING1B, whereas the catalytic component of PRC2, Ezh2, methylates lysine-27 of histone H3 (H3K27me2/3) in cooperation with other PRC2 components, such as Suz12 and Eed. Ezh2 has attracted intense interest not only because of its role in maintaining stemness, but also because its deregulation contributes to cancer [4] , [5] . Ezh2 is highly expressed in numerous human cancers, including breast and prostate, with the highest Ezh2 levels correlating with advanced stages of tumour progression and poor prognosis [6] . Moreover, mutation of Ezh2 Y641 has been described in lymphomas [7] and results in Ezh2 gain-of-function [8] , [9] . Oncogenic activity of Ezh2 has also been described in myelodysplastic syndromes [10] and in acute myeloid leukaemia [11] , where it has been identified as a potential drug target [12] . However, acquired Ezh2 mutations in myeloid neoplasms have also been found, indicating that Ezh2 may act as a tumour suppressor [13] , [14] . Thus, increases and decreases in the H3K27 methylation activity of Ezh2 may both lead to cancer. Understanding the role of Ezh2 in haematologic tumour progression requires the controlled manipulation of Ezh2 levels in vivo . In the present study, we generated mouse models that allow gain-of-function of Ezh2 in the haematopoietic system. Activation of Ezh2 expression specifically in self-renewing HSCs alters gene expression programs and severely compromises haematopoietic function, leading to the development of myeloproliferative disease. Expression of Ezh2 affects the HSC populations To investigate the effect of increased Ezh2-mediated H3K27 methylation in vivo , we generated conditional knock-in Ezh2 fl/fl mice (cki Ezh2 fl/fl ) by targeting a conditional construct encoding Ezh2 cDNA to the genomic ROSA26 locus ( Supplementary Fig. S1a ). To induce Ezh2 in the haematopoietic system, targeted transgenic cki Ezh2 fl/fl mice were bred with vav-Cre transgenic mice expressing Cre recombinase in haematopoietic cells [15] (hereafter referred to as Ezh2-KI and control) ( Supplementary Fig. S1b ). In Ezh2-KI mice, Ezh2 messenger RNA levels were 2–3 fold higher in thymus and in spleen ( P <0.05), and fourfold higher ( P <0.05) in bone marrow (BM) compared with control littermates ( Supplementary Fig. S2a ). As expected, increased Ezh2 protein levels were not only detected in spleen and LSKs from Ezh2-KI mice, but also correlated with increased H3K27me3 levels ( Supplementary Fig. S2b ). To test whether adverse effects of Cre activity contribute to the phenotype of transgenic Ezh2-KI mice, we intercrossed mice carrying the R26R-GFP reporter with vavCre tg/+ mice ( Supplementary Fig. S3a,b ). We detected green fluorescent protein (GFP) expression in LSKs, as well as in other haematopoietic fractions of R26R/Cre + mice ( Supplementary Fig. S3c ), consistently with previous studies using transgenic mice driving Cre expression from vav promoter [15] , [16] , [17] . Moreover, the total numbers of white blood cells (WBC), lymphocytes, monocytes, granulocytes, platelets and red blood cells were comparable between the two genotypes ( Supplementary Fig. S3d ). Together, these results indicate that Cre expression from the vav promoter does not of itself influence phenotype. To investigate the potential role of Ezh2 in regulating primitive haematopoietic cell function, we determined the haematopoietic subpopulation profile in BM. Compared with controls, BM of Ezh2-KI mice contained a significantly higher frequency and absolute number of long-term repopulating HSCs (LT-HSC; P <0.05) and short-term HSCs (ST-HSC; P <0.05), whereas this increase was exacerbated in aged mice (50-week-old; P <0.05; Supplementary Fig. S4a ). In contrast, the multipotent progenitor fraction (MPP) was proportionately and absolutely smaller ( Fig. 1a,b ). As the total number of mononuclear cells per femur was similar in the two genotypes ( Supplementary Fig. S2c ), these data indicate an increase in the absolute number of repopulating HSCs in targeted transgenic Ezh2-KI mice. 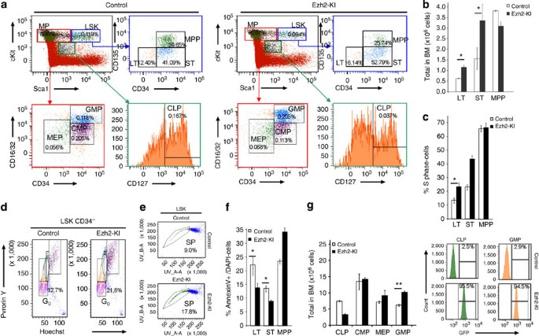Figure 1: Ezh2 gain-of-function in the haematopoietic lineage alters the HSC population profile in BM. (a) Representative FACS profiles of BM cells from Ezh2-KI mice and control littermates. FACS plots were gated on the L−S+K+(LSK) supopulation (blue gate), which was subclassified for expression of CD34 and CD135 to give the percentages of MPPs, and LT- and ST-HSCs. The CLP fraction was gated on LKlowSlowCD127+(green gate) expression. MP (red gate) were subclassified into CMP, GMP and MEP based on LKhighSnegCD16/32 and CD34 expression. At least six mice per genotype were tested, over at least two separate experiments. Numbers indicate percentages of the total nucleated BM cell population, except for the subclassification of LSK cells, where numbers indicate the percentage of the LSK subpopulation. (b) Absolute numbers per femur of the LT, ST and MPP primitive populations described in (a). Values are means±s.d. (n=12; *P<0.05). (c) Proliferation activity of LT, ST and MPP populations measured byin vivoBrdU incorporation over 48 h. Values are means±s.d. (n=10, *P<0.05). (d) FACS analysis of LSKCD34−cells in the quiescent G0phase of the cell cycle. Representative plots show Hoechst 33342 and PyroninY staining in control and Ezh2-KI mice. Numbers indicate the percentage of cells in G0from at least three independent experiments (P<0.05). (e) SP in LSK populations from control and Ezh2-KI mice, identified by Hoechst 33342 staining and the use of blue and red filters. Numbers indicate the percentage of SP cells from three independent experiments. (f) AnnexinV-DAPI analysis of the percentage of early apoptotic cells in the LSK subpopulations. Values are means±s.d. (*P<0.05;n=6). (g) Left: absolute numbers per femur of the CLP, CMP, MEP and GMP subpopulations (as described inFig. 1a) in BM from control and Ezh2-KI mice. Values are means±s.d. (n=10, **P<0.001). Right: representative FACS plots showing GFP expression in the total CLP and GMP subpopulations of Ezh2-KI and control mice. Numbers are the percentages of GFP+ cells from at least three independent experiments. The statistical significance of differences was measured by unpaired two-tailed Student'st-test: *P<0.05, **P<0.001. Figure 1: Ezh2 gain-of-function in the haematopoietic lineage alters the HSC population profile in BM. ( a ) Representative FACS profiles of BM cells from Ezh2-KI mice and control littermates. FACS plots were gated on the L − S + K + (LSK) supopulation (blue gate), which was subclassified for expression of CD34 and CD135 to give the percentages of MPPs, and LT- and ST-HSCs. The CLP fraction was gated on LK low S low CD127 + (green gate) expression. MP (red gate) were subclassified into CMP, GMP and MEP based on LK high S neg CD16/32 and CD34 expression. At least six mice per genotype were tested, over at least two separate experiments. Numbers indicate percentages of the total nucleated BM cell population, except for the subclassification of LSK cells, where numbers indicate the percentage of the LSK subpopulation. ( b ) Absolute numbers per femur of the LT, ST and MPP primitive populations described in ( a ). Values are means±s.d. ( n =12; * P <0.05). ( c ) Proliferation activity of LT, ST and MPP populations measured by in vivo BrdU incorporation over 48 h. Values are means±s.d. ( n =10, * P <0.05). ( d ) FACS analysis of LSKCD34 − cells in the quiescent G 0 phase of the cell cycle. Representative plots show Hoechst 33342 and PyroninY staining in control and Ezh2-KI mice. Numbers indicate the percentage of cells in G 0 from at least three independent experiments ( P <0.05). ( e ) SP in LSK populations from control and Ezh2-KI mice, identified by Hoechst 33342 staining and the use of blue and red filters. Numbers indicate the percentage of SP cells from three independent experiments. ( f ) AnnexinV-DAPI analysis of the percentage of early apoptotic cells in the LSK subpopulations. Values are means±s.d. (* P <0.05; n =6). ( g ) Left: absolute numbers per femur of the CLP, CMP, MEP and GMP subpopulations (as described in Fig. 1a ) in BM from control and Ezh2-KI mice. Values are means±s.d. ( n =10, ** P <0.001). Right: representative FACS plots showing GFP expression in the total CLP and GMP subpopulations of Ezh2-KI and control mice. Numbers are the percentages of GFP+ cells from at least three independent experiments. The statistical significance of differences was measured by unpaired two-tailed Student's t -test: * P <0.05, ** P <0.001. Full size image Ezh2 contributes to the self-renewing HSC maintenance To identify how Ezh2 maintains the stem cell compartment, we first analysed the cell-cycle frequency of Ezh2-KI primitive HSCs over 48 h. The percentage of BrdU-incorporating LT- and ST-HSCs was higher in Ezh2-KI mice than in counterpart controls ( Fig. 1c ). We also examined the cell-cycle status of the LSKCD34 − subpopulation and observed increased numbers of Pyrorin Y low cells, indicating a higher abundance of quiescent HSCs in Ezh2-KI mice ( P <0.05; Fig. 1d ). Analysis of LSK cells for the side population (SP) phenotype, a marker of quiescent HSCs in adult BM [18] , also revealed a twofold increase in LSK-SP cells in Ezh2-KI mice ( P =0.04; Fig. 1e ). Examination of the annexinV + /DAPI − population showed that the number of apoptotic LT- and ST-HSCs was lower in Ezh2-KI mice than in controls ( P <0.05), whereas the number of apoptotic MPP cells was higher in the knock-in mice ( P =0.04) ( Fig. 1f ). These data suggest that Ezh2 increases the pool of quiescent HSCs, by favouring their cell cycling and reducing apoptosis, while having opposite effects on the MPP pool. Ezh2-KI mice aberrantly prime to produce mature myeloid cells Analysis of GFP status in myeloid progenitor subpopulations of Ezh2-KI mice revealed a significant expansion only in the GMP population (94.5% of cells GFP + ; P <0.001; Fig. 1g ); and again this decrease was exacerbated in aged Ezh2-KI animals ( P <0.001; Supplementary Fig. S4a ). This population accounted for almost all of the increased numbers of myeloid progenitors (MP), with the numbers of common myeloid progenitor (CMP) and myeloid erythroid progenitor (MEP) remaining similar to control animals ( Fig. 1a,g ). Notably, Ezh2-KI mice showed a lower frequency of common lymphoid progenitors (CLP) than control animals ( Fig. 1g ). BrdU incorporation experiments revealed that GMPs from Ezh2-KI mice were more proliferative than their counterpart controls ( P =0.04), whereas CMP and MEP cells showed little difference between genotypes ( Fig. 2a ). 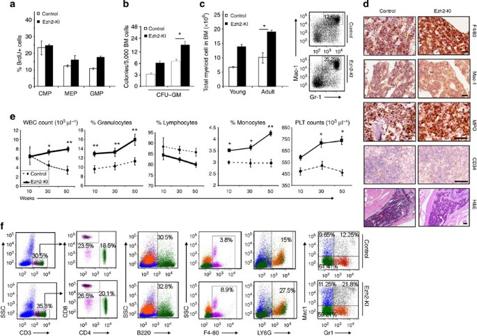Figure 2: Haematopoietic-specific transgenic Ezh2 expression induces myeloproliferation. (a) Proliferation activity of different myeloid progenitors (CMP, MEP and GMP) in BM was assessed using BrdU incorporationin vivoover 48 h. Values are means±s.d.,n=4. (b) Granulocyte–macrophage colony formation by BM cells from young (10-week-old) and adult (30-week-old) control and Ezh2-KI mice. Data are the numbers of live colonies (>30 cells) formed after 12 day culture on methylcellulose supplemented with granulocyte–macrophage colony stimulating factor (GM–CSF; 10 ng ml−1). Values are means±s.d. (n=10, *P<0.05). (c) Left: absolute numbers per femur of mature myeloid cell populations (Mac-1/Gr-1) in BM from control and Ezh2-KI mice. Values are means±s.d. (n=12, *P<0.05). Right: representative FACS plots showing the percentages of Mac-1+/Gr-1lowand Mac-1+/Gr-1+cells in Ezh2-KI and control animals from at least three independent experiments. (d) Histological and immunohistological characterization of BM sections from Ezh2-KI and control mice with H&E (×40 magnification), anti-MPO (×200 magnification), anti-F4-80 (×100 magnification), anti-CD34 (×200 magnification)and anti-Mac1 (×100 magnification) antibodies. The bar indicates 100 μm. (e) PB counts of Ezh2-KI and control mice at 10-, 30- and 50-week-old. PLT, platelets. Values are means±s.d. (n=8, *P<0.05; **P<0.001). (f) Representative FACS plots showing the percentages of lymphoid (CD3, CD4/CD8 and B220) and myeloid (Mac-1/Gr-1, F4-80 and Ly6G) -positive cells in Ezh2-KI and control animals (mean±s.d.;n=8; *P<0.05). The statistical significance of differences was measured by unpaired two-tailed Student'st-test: *P<0.05, **P<0.001. Figure 2: Haematopoietic-specific transgenic Ezh2 expression induces myeloproliferation. ( a ) Proliferation activity of different myeloid progenitors (CMP, MEP and GMP) in BM was assessed using BrdU incorporation in vivo over 48 h. Values are means±s.d., n =4. ( b ) Granulocyte–macrophage colony formation by BM cells from young (10-week-old) and adult (30-week-old) control and Ezh2-KI mice. Data are the numbers of live colonies (>30 cells) formed after 12 day culture on methylcellulose supplemented with granulocyte–macrophage colony stimulating factor (GM–CSF; 10 ng ml −1 ). Values are means±s.d. ( n =10, * P <0.05). ( c ) Left: absolute numbers per femur of mature myeloid cell populations (Mac-1/Gr-1) in BM from control and Ezh2-KI mice. Values are means±s.d. ( n =12, * P <0.05). Right: representative FACS plots showing the percentages of Mac-1 + /Gr-1 low and Mac-1 + /Gr-1 + cells in Ezh2-KI and control animals from at least three independent experiments. ( d ) Histological and immunohistological characterization of BM sections from Ezh2-KI and control mice with H&E (×40 magnification), anti-MPO (×200 magnification), anti-F4-80 (×100 magnification), anti-CD34 (×200 magnification)and anti-Mac1 (×100 magnification) antibodies. The bar indicates 100 μm. ( e ) PB counts of Ezh2-KI and control mice at 10-, 30- and 50-week-old. PLT, platelets. Values are means±s.d. ( n =8, * P <0.05; ** P <0.001). ( f ) Representative FACS plots showing the percentages of lymphoid (CD3, CD4/CD8 and B220) and myeloid (Mac-1/Gr-1, F4-80 and Ly6G) -positive cells in Ezh2-KI and control animals (mean±s.d. ; n =8; * P <0.05). The statistical significance of differences was measured by unpaired two-tailed Student's t -test: * P <0.05, ** P <0.001. Full size image To quantify the recombination rate in myeloid progenitors, we generated CFU–GM colonies in methylcellulose medium. Ezh2-positive colonies were hypersensitive to GM–CSF ( Fig. 2b ; data not shown), consistent with cell-autonomous signaling in Ezh2-expressing haematopoietic cells. The BM of Ezh2-KI mice also showed a marked presence of mature myeloid cells (Mac-1 + /Gr-1 low and Mac-1 + /Gr-1 + ) in both young and adult-mutant animals ( P <0.05; Fig. 2c ). Immunohistochemistry (IHC) using anti-myeloperoxidase (MPO) antibodies effectively highlighted granulocytic cells and some monocytes, whereas immunostaining for myeloid cells (Mac-1) and macrophages (F4-80) demonstrated an excess of monocytes and macrophages relative to the controls ( Fig. 2d ). Corroborating the flow cytometric analysis, BM sections immunostained with myeloid-specific markers showed that Ezh2-KI BM was dominated by myeloid cells ( Fig. 2d ). These increases in primitive haematopoietic cell populations and later stage myeloid progenitors suggest that Ezh2 overexpression promotes expansion both of HSCs and of the myeloid lineage. To test the homing capacity of haematopoietic progenitors in Ezh2-KI mice, we transplanted lineage-negative CD45.2 + cells into lethally irradiated wild-type (CD45.1 + ) mice. Homing of donor cells to BM of recipient animals was assessed by expression of CD45.2. Cells from Ezh2-KI mice homed to the BM of recipient mice at a higher frequency than cells from control mice ( P <0.05; Supplementary Fig. S4c ). Together, these data indicate that the proliferative haematopoietic progenitors from Ezh2-KI mice are constitutively mobilized and favour rapid expansion of the myeloid lineage to mature myeloid cells. Ezh2 expression induces myeloid-proliferative disorder Analysis of peripheral blood (PB) cell counts in young Ezh2-KI mice (10-week-old) revealed prominent increases relative to controls of circulating granulocytes ( P <0.001). and monocytes relative to controls ( P <0.05) ( Fig. 2e ; Supplementary Fig. S4d ). These increases were exacerbated in adult mice (30-week-old; P <0.001; Fig. 2e ) and sustained in aged animals (50-weeks-old; P <0.001; Fig. 2e ). White blood cell, lymphocyte, erythrocyte and platelet counts were normal in young animals ( Fig. 2e ; Supplementary Fig. S4d ). However, over time, adult Ezh2-KI mice strikingly increased these differences in WBC and platelets counts ( P <0.001; Fig. 2e ; Supplementary Fig. S4d ). Flow cytometry analysis revealed similar frequencies of B and T lymphocytes in the two genotypes ( Fig. 2f ), whereas the granulocyte and macrophage populations were threefold greater in Ezh2-KI animals, and mature myeloid cells (Mac-1 + /Gr-1 low and Mac-1 + /Gr-1 + ) were also significantly increased ( P <0.05; Fig. 2f ). Ezh2-KI mice showed a marked splenomegaly, and it was reflected in an increased proportion of mature myeloid cells (Mac-1 + /Gr-1 + ; F4-80 and Ly6G) ( P <0.05) ( Fig. 3a–d ), whereas an increased number of CLPs detected in spleen could not be accounted for by the fraction of lymphoid cells ( Supplementary Fig. S4e ). The enlarged spleens of Ezh2-KI mice contained abnormally high numbers of cells with the phenotypic characteristics of LSKs, CLPs and GMPs ( Fig. 3e ), providing further evidence of increased mobilization of progenitors and extramedullar haematopoiesis. Immunohistochemical staining of spleen sections with myeloid-specific markers (MPO, F4-80 and Mac-1) corroborated the hyperproliferation of myeloid cells already detected by fluorescence-activated cell sorting (FACS) analysis ( Fig. 3f ). Furthermore, Ezh2 and Ki-67 immunostaining of splenic sections revealed an increase in the numbers Ezh2 expressing and proliferating (Ki-67 + ) cells in Ezh2-KI animals, both in red pulp and lymphoid follicles ( Fig. 3f ). Together, by modulating Ezh2 expression in the haematopoietic system in vivo by intercrossing Ezh2 conditional gain-of-function mice with a haematopoietic-specific vav-Cre line, we found that self-renewing HSCs expressing Ezh2 leads to fatal myeloproliferative disorder (MPD) ( Fig. 3g ). 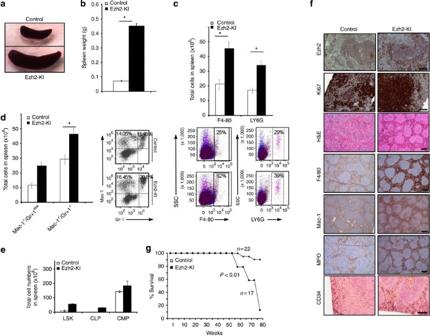Figure 3: Ezh2 expression induces myeloid-proliferative disorder. (a) Photograph of spleen from Ezh2-KI and control mice (50-week-old), showing splenomegaly in Ezh2-KI animals. (b) Spleen weight in Ezh2-KI and control mice. Values are means±s.d. (n=12, *P<0.05). (c) Top: absolute numbers of macrophages (F4-80) and granulocytes (LY6G) in spleen from control and Ezh2-KI mice. Values are means±s.d. (n=12, *P<0.05). Bottom: representative FACS plots showing the percentages of F4/80 and LY6G cells in the spleen from Ezh2-KI and control animals. (d) Left: absolute numbers of mature myeloid cell populations (Mac-1/Gr-1) in spleen from control and Ezh2-KI mice. Values are means±s.d. (n=12, *P<0.05). Right: representative FACS plots showing the percentages of Mac-1+/Gr-1lowand Mac-1+/Gr-1+cells in the spleen from Ezh2-KI and control animals. (e) Absolute numbers of LSK, CLP and CMP populations in spleen from Ezh2-KI and control mice. Values are means±s.d. (n=12). (f) Histological and immunohistological characterization of spleen sections from Ezh2-KI and control mice with H&E (×40 magnification), and anti-Ezh2 (100× magnification), anti-Ki67 (×100 magnification), anti-MPO (×40 magnification), anti-F4-80 (×40 magnification), anti-CD34 (×40 magnification), and anti-Mac1 (×40 magnification) antibodies. The bar indicates 100 μm. (g) Kaplan–Meier survival plot showing survival rates for Ezh2-KI mice or littermate controls (*P<0.001). The statistical significance of differences was measured by unpaired two-tailed Student'st-test: *P<0.05, **P<0.001. Figure 3: Ezh2 expression induces myeloid-proliferative disorder. ( a ) Photograph of spleen from Ezh2-KI and control mice (50-week-old), showing splenomegaly in Ezh2-KI animals. ( b ) Spleen weight in Ezh2-KI and control mice. Values are means±s.d. ( n =12, * P <0.05). ( c ) Top: absolute numbers of macrophages (F4-80) and granulocytes (LY6G) in spleen from control and Ezh2-KI mice. Values are means±s.d. ( n =12, * P <0.05). Bottom: representative FACS plots showing the percentages of F4/80 and LY6G cells in the spleen from Ezh2-KI and control animals. ( d ) Left: absolute numbers of mature myeloid cell populations (Mac-1/Gr-1) in spleen from control and Ezh2-KI mice. Values are means±s.d. ( n =12, * P <0.05). Right: representative FACS plots showing the percentages of Mac-1 + /Gr-1 low and Mac-1 + /Gr-1 + cells in the spleen from Ezh2-KI and control animals. ( e ) Absolute numbers of LSK, CLP and CMP populations in spleen from Ezh2-KI and control mice. Values are means±s.d. ( n =12). ( f ) Histological and immunohistological characterization of spleen sections from Ezh2-KI and control mice with H&E (×40 magnification), and anti-Ezh2 (100× magnification), anti-Ki67 (×100 magnification), anti-MPO (×40 magnification), anti-F4-80 (×40 magnification), anti-CD34 (×40 magnification), and anti-Mac1 (×40 magnification) antibodies. The bar indicates 100 μm. ( g ) Kaplan–Meier survival plot showing survival rates for Ezh2-KI mice or littermate controls (* P <0.001). The statistical significance of differences was measured by unpaired two-tailed Student's t -test: * P <0.05, ** P <0.001. Full size image Comparable in vivo and in vitro phenotypes were seen using a second model system in which Ezh2 was overexpressed using the tamoxifen-inducible Rosa26 Cre-ER T2 mice [19] (hereafter termed Ezh2-KI-ER) ( Supplementary Fig. S5a-g ). Together, these results show that inducible Ezh2 gain-of-function induces the proliferation of haematopoietic progenitors and initiates a myeloproliferative disease similar to that observed in constitutive Ezh2-KI mice. Myeloid-restricted Ezh2 expression does not generate MPD To identify the developmental stage at which activation of Ezh2 leads to MPD, we crossed cki Ezh2 fl/fl mice with mice bearing the lysozyme-M Cre (LyzMCre) recombinase transgene [20] , allowing expression of Ezh2 in the myeloid lineage. More than 70% of granulocytes in 8-week-old Ezh2 fl/fl /Cre-M tg/+ mice (Ezh2-KI-M) were GFP + ( Supplementary Fig. S6a ). Consistent with this, increased Ezh2 expression was detected in a subset of myeloid progenitors and in macrophages, platelets, monocytes and significantly in granulocytes ( P <0.05) ( Supplementary Fig. S6b ). PB of control and Ezh2-KI-M mice contained comparable amounts of leukocytes, platelets, red blood cells and haemoglobin ( Supplementary Fig. S6c ). Numbers of GMPs and granulocytes were slightly higher in BM of Ezh2-KI-M mice, but there was no significant expansion of the granulocytic population in spleen ( Supplementary Fig. S6d,e ). Moreover, relative numbers of myeloid cells did not increase further during the 10-month observation period and animals did not develop MPD. Therefore, targeted Ezh2 expression in the myeloid lineage does not induce MPD. Ezh2 contributes to the repopulating ability of HSCs The long-term engraftment potential of haematopoietic cells is predominantly a property of LT-HSCs [21] . Given that Ezh2-KI mice produced more repopulating HSCs than controls, we investigated their reconstitution properties. BM cells from 8-week-old control and Ezh2-KI mice (CD45.2) were transplanted in competition (1:1 and 1:10) with wild-type CD45.1 cells, and analysed 16 weeks after transplantation ( Fig. 4a ). Ezh2-KI donor cells, but not counterpart controls, strikingly outcompeted CD45.1 + competitor cells ( P <0.05) ( Fig. 4b,c ). This is probably due, in part, to the enrichment of stem cells in the Ezh2-KI donor population, but may also reflect the higher proliferation capacity of this population. BrdU incorporation at the end of the 16-week period confirmed that donor cells from Ezh2-KI mice cycled more rapidly than controls ( Fig. 4d ). This change in cell cycling by Ezh2 knock-in cells was consistent with the findings described in Figure 1c . Moreover, the recipients of Ezh2-KI and controls showed no significant differences in the percentage of apoptotic cells in primitive BM populations ( Fig. 4e ). Therefore, the increase in stem-cell number and function in Ezh2-KI animals was associated with a combination of higher cycling activity and a lower frequency of cell death. Moreover, PB contained a significantly higher fraction of white blood cells ( Fig. 4f ) and mature myeloid cells originating from Ezh2-KI donors ( P <0.001; Fig. 4g ). In BM, Ezh2-KI cells made a bigger contribution to primitive (LSK) repopulating populations and to myeloid and lymphoid progenitors ( Fig. 4h ). 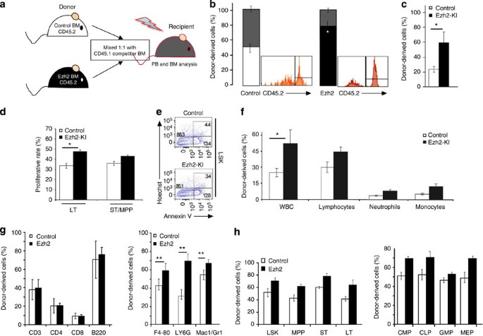Figure 4: Functional impact of the Ezh2 overactivity on BM reconstitution. (a) Scheme of the competitive repopulation assay. At 16 weeks post transplant, BM and PBPB cells were analysed for donor-derived (CD45.2) contribution. (b,c) Average chimerism in post-transplant competitive recipients translplanted with 1:1 (b) and 1:10 (c) ratios of donor and competitor cells, analysed by the contribution of donor-derived (CD45.2) cells to PB. Values are means±s.d. (n=10, *P<0.05). (d) Proliferation rate of BM LT-HSC and ST-HSC/MPP populations from recipient mice measured byin vivoBrdU incorporation over 24 h. Column figures show proliferation rate (%), where values are the means±s.d. (n=6, *P<0.05). (e) AnnexinV-Hoechst analysis of the percentage of early apoptotic cells in the LSK subpopulation of recipient mice. Values are means±s.d. (n=8). (f) FACS analysis of the contribution of donor-derived cells to white blood cells (WBC), lymphocytes, monocytes and neutrophils in PB of transplant recipients. The bar graph shows the percentages (mean±s.d.) of the indicated populations in PB (n=7, *P<0.05). (g,h) Average chimerism in post-transplant recipients analysed by the contribution of donor-derived (CD45.2) BM cells to the circulating fractions of (g) mature myeloid (Mac-1/Gr-1), macrophages (F4-80) and granulocytes (LY6G); and (h) primitive HSCs subfractions, and CLP, CMP, MEP and GMP progenitors in transplant recipients. Values are means±s.d. (n=8; **P<0.001). The statistical significance of differences was measured by unpaired two-tailed Student'st-test: *P<0.05, **P<0.001. Figure 4: Functional impact of the Ezh2 overactivity on BM reconstitution. ( a ) Scheme of the competitive repopulation assay. At 16 weeks post transplant, BM and PBPB cells were analysed for donor-derived (CD45.2) contribution. ( b , c ) Average chimerism in post-transplant competitive recipients translplanted with 1:1 ( b ) and 1:10 ( c ) ratios of donor and competitor cells, analysed by the contribution of donor-derived (CD45.2) cells to PB. Values are means±s.d. ( n =10, * P <0.05). ( d ) Proliferation rate of BM LT-HSC and ST-HSC/MPP populations from recipient mice measured by in vivo BrdU incorporation over 24 h. Column figures show proliferation rate (%), where values are the means±s.d. ( n =6, * P <0.05). ( e ) AnnexinV-Hoechst analysis of the percentage of early apoptotic cells in the LSK subpopulation of recipient mice. Values are means±s.d. ( n =8). ( f ) FACS analysis of the contribution of donor-derived cells to white blood cells (WBC), lymphocytes, monocytes and neutrophils in PB of transplant recipients. The bar graph shows the percentages (mean±s.d.) of the indicated populations in PB ( n =7, * P <0.05). ( g , h ) Average chimerism in post-transplant recipients analysed by the contribution of donor-derived (CD45.2) BM cells to the circulating fractions of ( g ) mature myeloid (Mac-1/Gr-1), macrophages (F4-80) and granulocytes (LY6G); and ( h ) primitive HSCs subfractions, and CLP, CMP, MEP and GMP progenitors in transplant recipients. Values are means±s.d. ( n =8; ** P <0.001). The statistical significance of differences was measured by unpaired two-tailed Student's t -test: * P <0.05, ** P <0.001. Full size image To exclude an effect of Ezh2 expression in the BM microenvironment on adult haematopoiesis, we transplanted wild-type BM cells (CD45.1) into lethally irradiated Ezh2-KI or littermate control mice (CD45.2). Examination of PB and BM revealed no differences in engraftment between genotypes at all time points examined ( Supplementary Fig. S7a,b ), indicating that the Ezh2-KI microenvironment does not influence the engraftment of HSCs. Taken together, these results suggest that Ezh2-expressing repopulating HSC subpopulations are highly efficient at long-term repopulation, and give rise to significantly increased levels of mature myeloid cells in recipient animals. Ectopic Ezh2 on BM cells is haematopoietic cell autonomous To investigate the cell-intrinsic nature of the phenotypic defects of Ezh2-KI mice, we tested the ability of unfractioned Ezh2-KI BM cells to reproduce these defects in wild-type CD45.1 recipients. After secondary transplantation with Ezh2-KI BM cells, which yielded a high percentage of chimerism ( Fig. 5a ), lethally irradiated recipient mice began to develop MPD, characterized at 10 weeks by progressive enlargement of spleens ( Fig. 5b ) and increased numbers of monocytes ( P <0.001), platelets ( P <0.05), and granulocytes ( P <0.05) ( Table 1 ). This was followed at 16 weeks post transplantation by substantial increases in total WBC counts ( Fig. 5c ). Moreover, second transplanted BM cells formed bigger and high colonies in in vitro colony-forming assays ( Fig. 5d ). FACS analysis confirmed increased numbers myeloid cells ( P <0.05) originating from Ezh2-KI donor, and showed that lymphoid populations were unaffected ( Fig. 5e ). Thus, secondary recipient mice manifest a progressive MPD similar to that seen in the original Ezh2-KI donors. Strikingly, after the third transplant cycle, recipients of Ezh2-KI cells died by week 2–4 post transplant by developing aggressive MPD ( P <0.01; Fig. 5f ), whereas recipients of control cells survived; lethally irradiated animals that did not receive BM transplant ( n =4) survived 10–14 days (data not shown). Lineage contribution analysis suggested that the effect of this third serial transplantation was primarily attributable to excess expansion of myeloid cells from secondary transplants Ezh2-KI BM cells, marked by elevated myeloid presence in BM and spleen of mature myeloid cells ( Fig. 5g ). To determine whether increased cytokine sensitivity in these tertiary transplanted animals also occurred at the level of stem cell/progenitors, LSK cells were cultured in the presence of IL-3. Tertiary-transplanted Ezh2-overexpressing cells were increased 100-fold, compared with a 30-fold increase for wild-type cells ( Supplementary Fig. S7c ), indicating that the accompanying myeloid differentiation induced by this cytokine was enhanced by Ezh2. These results verify the cell-autonomous effect of Ezh2 on sensitizing HSCs/progenitors to cytokine-induced differentiation. Together, these data suggests that the effect of Ezh2 overexpression on HSCs is haematopoietic cell autonomous. 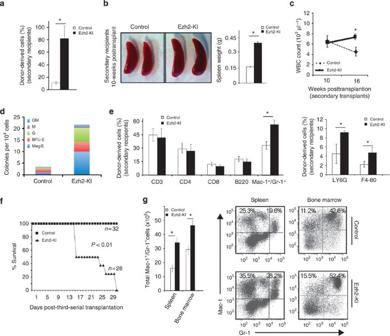Figure 5: Ezh2 function in haematopoiesis is cell autonomous. (a) Average chimerism in post-transplant secondary recipients analysed by the contribution of donor-derived (CD45.2) cells to PB (separated by a 10-week reconstitution period). Values are means±s.d. (n=12, *P<0.05). (b) Photographs and weights of spleens from Ezh2-KI and control mice demonstrating progressive splenomegaly in secondary recipient mice transplanted with BM from Ezh2-KI or donors, 16 weeks post-transplant. (c) PB counts in recipients after secondary transplant at 10 (c) and 16 (d) weeks post transplant . Values are means±s.d. (n=8, *P<0.05). (d) CFU-C assay using BM cells prepared, as indicated in Methods Section. Cells from at least three secondary recipients per genotype were plated in triplicate, and colonies were scored 7 days later. The graph represents the means of total colonies from duplicate cultures. Similar results were obtained with three different pairs of control and Ezh2-KI mice. Meg/E, megakaryocyte/erythroid colonies; BFU-E burst formation unit-erythroid; G, granulocyte colonies; M, macrophage colonies; GM, granulocyte/macrophage colonies; GEMM, granulocyte, erythroid, macrophage and megakaryocyte colonies. (e) Average of chimerism in post-transplant secondary recipients analysed for the contribution of donor-derived (CD45.2) cells in BM for circulating mature myeloid (Mac-1/Gr-1), macrophages (F4-80) and granulocytes (LY6G) (G); and lymphoid subfractions (CD3, CD4, CD8 and B220) in transplant recipients. Values are means±s.d. (n=8; *P<0.05). (f) Kaplan–Meier survival plot showing survival rates for tertiary recipients of BM originating from Ezh2-KI mice or littermate controls. (g) Right: absolute numbers of mature myeloid cell populations (Mac-1/Gr-1) in the spleen and BM of tertiary recipients of BM originating from Ezh2-KI mice or littermate controls. Values are means±s.d. (n=12, *P<0.05). Left: representative FACS plots showing the percentages of Mac-1+/Gr-1lowand Mac-1+/Gr-1+cells in Ezh2-KI and control animals (n=4). The statistical significance of differences was measured by unpaired two-tailed Student'st-test: *P<0.05, **P<0.001. Figure 5: Ezh2 function in haematopoiesis is cell autonomous. ( a ) Average chimerism in post-transplant secondary recipients analysed by the contribution of donor-derived (CD45.2) cells to PB (separated by a 10-week reconstitution period). Values are means±s.d. ( n =12, * P <0.05). ( b ) Photographs and weights of spleens from Ezh2-KI and control mice demonstrating progressive splenomegaly in secondary recipient mice transplanted with BM from Ezh2-KI or donors, 16 weeks post-transplant. ( c ) PB counts in recipients after secondary transplant at 10 ( c ) and 16 ( d ) weeks post transplant . Values are means±s.d. ( n =8, * P <0.05). ( d ) CFU-C assay using BM cells prepared, as indicated in Methods Section. Cells from at least three secondary recipients per genotype were plated in triplicate, and colonies were scored 7 days later. The graph represents the means of total colonies from duplicate cultures. Similar results were obtained with three different pairs of control and Ezh2-KI mice. Meg/E, megakaryocyte/erythroid colonies; BFU-E burst formation unit-erythroid; G, granulocyte colonies; M, macrophage colonies; GM, granulocyte/macrophage colonies; GEMM, granulocyte, erythroid, macrophage and megakaryocyte colonies. ( e ) Average of chimerism in post-transplant secondary recipients analysed for the contribution of donor-derived (CD45.2) cells in BM for circulating mature myeloid (Mac-1/Gr-1), macrophages (F4-80) and granulocytes (LY6G) (G); and lymphoid subfractions (CD3, CD4, CD8 and B220) in transplant recipients. Values are means±s.d. ( n =8; * P <0.05). ( f ) Kaplan–Meier survival plot showing survival rates for tertiary recipients of BM originating from Ezh2-KI mice or littermate controls. ( g ) Right: absolute numbers of mature myeloid cell populations (Mac-1/Gr-1) in the spleen and BM of tertiary recipients of BM originating from Ezh2-KI mice or littermate controls. Values are means±s.d. ( n =12, * P <0.05). Left: representative FACS plots showing the percentages of Mac-1 + /Gr-1 low and Mac-1 + /Gr-1 + cells in Ezh2-KI and control animals ( n =4). The statistical significance of differences was measured by unpaired two-tailed Student's t -test: * P <0.05, ** P <0.001. Full size image Table 1 Peripheral blood counts in recipients after secondary transplant at 10 weeks post transplant and in recipients 4- and 12-week-post transplants with sorted LT/ST-HSCs. Full size table The MPD of Ezh2-KI mice is induced by Ezh2-KI HSCs To identify which BM subpopulation is responsible for the transfer of MPD to secondary recipients, we injected lethally irradiated wild-type CD45.1. mice with highly purified subpopulations isolated from 18-week-old Ezh2-KI mice. Injection of a mix of CMPs, GMPs and MEPs contributed less than 5% of circulating myeloid cells in primary recipients one month after transplantation, irrespective of Ezh2 expression ( Fig. 6a ). In contrast, injection of LT- and ST-HSCs from Ezh2-KI animals triggered mild-to-moderate myeloproliferation ( Fig. 6b ), manifested by a marked increase in myeloid cell number in PB ( Table 1 ), an effect also evidenced by increased WBC counts over time ( Table 1 ). Thus LT- and ST-HSCs are uniquely able to transplant the MPD observed in primary Ezh2-KI donor mice, indicating that the haematopoietic phenotype associated with Ezh2 expression is specifically induced by primitive haematopoietic populations. The transplantability of MPD, especially in recipients transplanted with LT- and ST-HSCs, supports the idea that the pathogenic effects of Ezh2-everexpressing cells are cell autonomous. 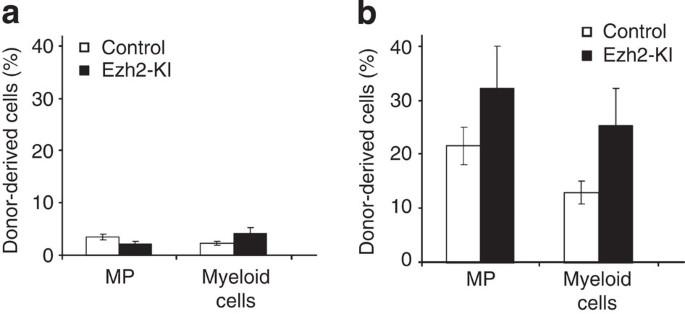Figure 6: HSCs but not myeloid progenitors from Ezh2-KI mice induces MPD in recipient hosts. (a,b) Subpopulation profiles in BM (myeloid progenitors, MP) and PB (mature myeloid cells, Mac-1+/Gr-1+) of recipient mice transplanted with either (a) pooled myeloid progenitors (Lin−c-kit+Sca-1−) or (b) LT/ST-HSCs from Ezh2-KI or control donors. Values are means±s.d.,n=4 recipients per group. Similar results were obtained in a second experiment. Figure 6: HSCs but not myeloid progenitors from Ezh2-KI mice induces MPD in recipient hosts. ( a , b ) Subpopulation profiles in BM (myeloid progenitors, MP) and PB (mature myeloid cells, Mac-1 + /Gr-1 + ) of recipient mice transplanted with either ( a ) pooled myeloid progenitors (Lin − c-kit + Sca-1 − ) or ( b ) LT/ST-HSCs from Ezh2-KI or control donors. Values are means±s.d., n =4 recipients per group. Similar results were obtained in a second experiment. Full size image Regulation of HSC-maintenance genes by Ezh2 Given the broad role of PCR2 family proteins as chromatin repressors, we conducted a global gene expression analysis of Ezh2-expressing LSKs to identify the most direct targets of Ezh2. Analysis of gene arrays using stringent criteria identified a specific Ezh2 signature in Ezh2-KI LSK cells. The most significantly up- and down-regulated genes are depicted in Supplementary Figure S8a . A complete list of all differentially regulated genes has been deposited in the Gene Expression Omnibus under accession no. GSE28369 , and summarized as a heat map presentation in Supplementary Figure S8b . Enriched expression was observed for several genes encoding extracellular proteins implicated in HSC quiescence [22] , including biglycan (BGN) [23] and angiopoietin 1 (ANGPT1) [24] , whereas NTRK3, important oncogenic tyrosine kinase in haematologic malignancies [25] , was downregulated. We also observed significant Ezh2-mediated expression of master transcriptional regulators of HSC-specific genes [26] , for example, EVI-1, ATF4 and IKZF1, essential molecular markers in leukaemias [27] , [28] . In addition to its DNA-binding activity, EVI-1 can recruit proteins, including histone methyl transferases [29] , to generate complexes for transcriptional regulation. The differential expression of several of the genes enriched in Ezh2-expressing LSKs from Ezh2-KI mice was validated by quantitative RT–PCR (qRT–PCR) ( Fig. 7a ). qRT–PCR showed the same trend in Ezh2-KI LSK cells seen in array analysis, with increased expression of EVI-1 , BGN , ANGPT1 and decreased expression of NTRK3 , ATF4 and IKZF1 . 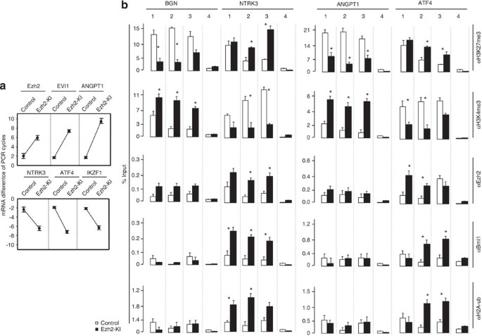Figure 7: Ezh2 signature in Ezh2-KI LSK cells. (a) Expression of totalEZH2,EVI-1,BGN,ANGPT1,NTRK3,ATF4ORIKZF1mRNA was measured in the sorted LSK subpopulation from control and Ezh2-KI mice by qRT–PCR. Results are normalized to β-actin expression and are expressed as difference of PCR cycles (means±s.d.;n=4). (b) ChIP analysis ofBGN,NTRK3,ANGPT1andATF4promoter regions in control and Ezh2-KI lineage−cells with antibodies to H3K27me3, H3K4me4, Ezh2, Bmi1 and H2A-ub. Primer sets 1–3 indicate different locations in the promoter regions, and set 4 indicates non-promoter amplified regions. Percentages of input DNA are shown as the means±s.d. of triplicate independent experiments (*P<0.05). The statistical significance of differences was measured by unpaired two-tailed Student'st-test: *P<0.05. Figure 7: Ezh2 signature in Ezh2-KI LSK cells. ( a ) Expression of total EZH2 , EVI-1 , BGN , ANGPT1 , NTRK3 , ATF4 OR IKZF1 mRNA was measured in the sorted LSK subpopulation from control and Ezh2-KI mice by qRT–PCR. Results are normalized to β-actin expression and are expressed as difference of PCR cycles (means±s.d. ; n =4). ( b ) ChIP analysis of BGN , NTRK3 , ANGPT1 and ATF4 promoter regions in control and Ezh2-KI lineage − cells with antibodies to H3K27me3, H3K4me4, Ezh2, Bmi1 and H2A-ub. Primer sets 1–3 indicate different locations in the promoter regions, and set 4 indicates non-promoter amplified regions. Percentages of input DNA are shown as the means±s.d. of triplicate independent experiments (* P <0.05). The statistical significance of differences was measured by unpaired two-tailed Student's t -test: * P <0.05. Full size image To determine whether Ezh2 regulates the expression of genes selectively enriched in HSCs from Ezh2-KI mice, we performed chromatin immunoprecipitation (ChIP) assays. Ezh2 expression increased the amount of bound H3K27me3 in the promoter regions of NTRK3 and ATF4 , but not the BGN and ANGPT1 promoters ( Fig. 7b ; Supplementary Fig. S9 ). Moreover, examination of the specific binding of Ezh2 by ChIP assay using Ezh2-specific antibodies detected site-specific binding of Ezh2 to the promoter regions of NTRK3 and ATF4 and the INK4 / ARF locus [30] in Ezh2-KI cells, but not to the BGN and ANGPT1 promoters ( Fig. 7b ; Supplementary Fig. S10 ). These studies revealed direct association of Ezh2 with NTRK3 , ATF4 or INK4/ARF transcripts, whereas attenuated levels of Ezh2 protein and the H3K27me3 mark associated with BGN or ANGPT1 may contribute to increased BGN and ANGPT1 expression. We next assessed whether the upregulated BGN and ANGPT1 transcript expression in HSCs of Ezh2-KI mice resulted in changes in Polycomb-dependent histone modifications. As well as examining the level of the essential PRC1 member Bmi1, we examined the level of H2A ubiquitylation (H2A-ub), a histone modification mediated by PRC1 (ref. 31 ). The entire promoter regions of the downregulated NTRK3 and ATF4 genes in Ezh2-KI Lin − cells were significantly enriched for the H2A-ub signal and Bmi1, showing that the signal was probably specific. In contrast, the H2A-ub signal and Bmi1 were absent from the BGN and ANGPT1 promoters in Ezh2-KI Lin − cells, suggesting that Ezh2 action likely requires the binding of Bmi1 ( Fig. 7b ). To confirm the assembly of Ezh2, knockdown of Ezh2 reduced not only binding of Ezh2 and trimethylation of H3K27 at the promoter region of ARF4 , but also Bmi1-binding and H2A ubiquitylation signal ( Supplementary Fig. S11 ). In contrast, Bmi1 and H2A-ub signals at the ANGPT1 promoter were not altered, suggesting that Ezh2 is required for the binding of Bmi1. To further examine whether the DNA methylation status might account for the different expression states of the genes and differing effects of increasing Ezh2 levels, bisulfite sequencing detected minimal basal DNA methylation in the NTRK3 and ATF4 promoters of young Ezh2-KI LSKs cells ( Supplementary Fig. S12 ), although this DNA methylation was increased when aged Ezh2-KI cells were analysed (50-week-old) ( Supplementary Fig. S13 ). Together, these gene expression data strongly correlate with the haematopoietic phenotype of Ezh2-KI mice and indicate that regulation of NTRK3 and ATF4 on Ezh2 overexpression in LSK cells may prime these primitive haematopoietic stem cells to generate MPD in these mice. Here we report that the histone methyltransferease Ezh2 appears to have a key role in controlling homeostasis of the haematopoietic stem cell compartment. By modulating Ezh2 expression in the haematopoietic system in vivo by intercrossing Ezh2 conditional gain-of-function mice with a haematopoietic-specific vav-Cre line, we found that self-renewing HSCs expressing Ezh2 lead to MPD [32] , [33] . MPD was also observed in inducible Ezh2-KI-ER mice, in which we could control the timing of Ezh2 expression by injection with tamoxifen. Notably, targeted activation of Ezh2 in myeloid cells in the Ezh2-KI-M mice only mildly influences the homeostasis of the granulocytic lineage and never leads to MPD. The results presented here provide the first experimental demonstration of altered HSC function caused by overactive Ezh2 function, leading to MPD. Our mouse models of controlled Ezh2 expression indicate that haematological disorders induced by Ezh2 overexpression developed fatal MPD, characterized by excessive myeloid expansion in BM and spleen, elevated white blood cell counts and mature myeloid cells, and splenomegaly. Moreover, analysis of BM and spleen cells revealed heightened sensitivity of haematopoietic progenitor cells to cytokines in vitro . Taken together, these findings support a model in which Ezh2-mediated H3K27me3 induces MPD. Once Ezh2 protein has enacted its direct repressive effect through H3K27 methylation, full repression seems to require the subsequent action of other Polycomb members, as others have reported [31] . Our results, while validating only a small proportion of Ezh2-regulated transcripts, shed light on this matter, and contrast the binding of Ezh2 and Bmi1 to upregulated BGN and ANGPT1 genes. The action of Ezh2 might involve the action of other chromatin targets, such that activation or repression of a gene program by histone methylation closely synchronizes with other epigenetic adjustments, enabling fine regulation of cell specification processes. These data provide a starting point for further studies to uncover the underlying mechanisms of Ezh2-mediated haematopoiesis and probably leukaemogenesis. Recent studies have demonstrated that Ezh2 can bind to DNA methyltransferases, which can result in DNA methylation [34] , and that H3K27 methylation is prerequisite for de novo methylation [5] , [34] . Thus, oncogenic Ezh2 action marks genes that are prone to cancer-specific DNA methylation [35] , [36] . In cancer risk states, with abnormal regulation of tissue renewal, such tight transcriptional repression may favour the abnormal expansion of stem and progenitor cell populations [37] . This expansion may, in turn, select mutations in oncogenic genes, helping to promote abnormal growth and progression to invasiveness and malignancy [38] . Consistent with this idea, mutations in genes involved in the epigenetic regulators have recently been documented. Inactivating mutations for Ezh2 have been found in a large cohort of myeloid neoplasms and lymphomas [7] , [13] , [14] , [39] , although follow-up studies have revealed that several of those mutations actually lead to increased levels of H3K27me3 (refs 8 , 9 ). The question now is whether or not these mutations are critical drivers of the underlying myeloproliferative process or if some of the mutations are simply markers of cancer-associated genomic instability. Larger studies, incorporating detailed analyses, will be needed to further clarify the spectrum and frequency of mutations, the functional consequences of these mutations, the degree of genotypic overlap, and their clinical significance, particularly in predicting outcomes for available therapies. Our working model proposes a molecular progression during tumorigenesis that starts with abnormal expansion of Ezh2-expressing haematopoietic stem or myeloid progenitor cell compartments, in which genes such as ATF4 and NTRK3 undergo Ezh2-mediated gene silencing associated with progressive DNA methylation of their promoter CpG islands. In early stage cancer, with abnormal expansion of stem and progenitor cell populations, such epigenetic changes might result in mutations that affect expression or function of essential DNA methyltransferases, such as Ezh2 or other epigenetically relevant proteins, compounding the cancer-associated genomic instability [40] . Identification of cellular pools with the capacity to start the neoplastic transformation underlying MPD could allow a more rational classification and prognosis of disease and, eventually, the development of targeted therapy. In general, mouse models of MPD [41] , [42] have had limited success in recognizing the MPD-initiating cell population because of complexity in transplanting and reproducing the consequences of the primary disease [43] , [44] , [45] . Our results show that at least two distinct cellular subfractions, the Ezh2-KI LT- and ST-HSCs, are essential for MPD pathogenesis. The identification of Ezh2-activated LT- and ST-HSCs as potential leukaemic stem cells (LSCs) for the Ezh2-induced MPD lends further support to the notion that leukaemias and cancers may be sustained by rare LSCs or cancer stem cells [46] ( Supplementary Fig. S14 ). Because the only self-renewing capacity is sustained by the HSCs, we expect that only clones of Ezh2-expressing HSCs can induce and accumulate the epigenetic changes required for the progression and development to leukaemia. Future investigation of the stem cell-specific oncogenic role of Ezh2 in myeloid disorders should therefore provide a better molecular understanding of Ezh2-expressing HSCs acting with LSC functions. Mice The generation of cki- Ezh2 fl/+ mice, carrying the conditional ROSA26-Ezh2 allele, is described in Supplementary Information . The vav -Cre, Rosa26Cre-ER T2 and LyzM -Cre mouse lines, which were crossed with cki- Ezh2 fl/fl to generate Ezh2-KI ( Ezh2 fl/fl /vavCre tg/+ ), Ezh2-KI-ER ( Ezh2 fl/fl /Cre-ER tg/tg ) and Ezh2-KI-M ( Ezh2 fl/fl /LyzMCre tg/+ ) mice, respectively, were all generated after backcrossing two generations to C57BL/6. In addition, R26R reporter mice were crossed with Ezh2 +/+ -Cre tg/+ to generate R26R/Cre + and R26R/Cre − . All genotyping primers are listed in Supplementary Table S1 . In Ezh2-KI-ER mice, Cre was induced by injections on 5 consecutive days of 1 mg tamoxifen (Sigma) in corn coil. PB samples ( ∼ 50 μl) were collected by tail bleeding into tubes containing EDTA, and white blood cells, lymphocytes, monocytes, platelets and granulocytes were counted using a Hemavet 950FS cell counter (Drew Scientific). Wild-type C57BL/6 (CD45.2+) and C57BL6/SJL (CD45.1+) mice were purchased from The Jackson Laboratory. Ezh2-KI, Ezh2-KI-ER and Ezh2-KI-M mice were all on the C57BL/6, CD45.2 background, and were bred in-house. All mice were maintained in a pathogen-free environment, and were provided with standard care and nutrition according to institutional guidelines and animal study proposals approved by the CNIC. Transplantation assays Cells were transplanted into the congenic CD45.1 + . B6.SJL mouse strain and monitored for the presence of CD45.2 + donor-derived cells. For competitive transplants, 5×10 5 BM cells from individual Ezh2-KI or littermate mice (CD45.2) were transplanted together with 5×10 5 competitor cells (CD45.1) lethally irradiated (10Gy) 8-week-old B6.SJL mice (CD45.1). Repopulation was assessed at 16 weeks by FACS analysis of PB and BM. Noncompetitive serial transplants were initiated by transplanting 2×10 6 whole BM cells pooled from three control or Ezh2-KI donors (CD45.2) into each irradiated recipient (CD45.1). Secondary and tertiary transplants were performed after a 10-week engraftment period by pooling whole BM cells from 2 reconstituted recipients and transplanting 2×10 6 of these cells into new groups of 8 irradiated CD45.1 recipients. PB cells were obtained by tail vein nicking 10 or 16 weeks post transplantation. For homing assays, 5×10 6 CD45.2 cells from BM of individual Ezh2-KI and littermate mice were transplanted into lethally irradiated B6.SJL mice (CD45.1). BM cells were collected after 24 h and analysed by FACS. Flow cytometry and cell sorting Flow cytometry was performed as described [47] . Single-cell suspensions were prepared from BM, PB or spleen, and red cells were lysed with ACK buffer (NH 4 Cl/KHCO 3 ). Cells were analysed with a cocktail of biotinylated anti-mouse antibodies to Ly-6G, F4-80, CD3var epsilon, CD4, CD8a (Ly-2) and B220 (CD45R) (558451; BD Biosciences; according to the manufacturer's instructions). Cells were detected and sorted using streptavidin conjugated to Alexa647, APC/Alexa750, Q-dot605, 405 (Invitrogen), or R/PE (BD Biosciences) (these antibodies were used at 1:100). Directly conjugated antibodies used were as follows: cKit-PerCP/Cy5.5, cKit-PE, cKit-APC (CD117) and Flk2-PE (CD135) (BD Biosciences); Sca1-PE/Cy7, Sca1-APC and Sca1-PE (Ly 6A/E, Caltag); Ki-67-APC and Ki-67-Alexa647; and CD34-Alexa647, CD127-PE and CD16/32-Alexa700 (these antibodies were used at 1:100). PB cell counts were obtained by tail vein nicking, red blood cells were lysed with NH 4 Cl, and the remaining cells were stained with either APC-anti-CD45.2 (eBioscience) and PE/Cy5.5-anti-CD45.1 (eBioscience) and the following lineage surface markers: CD3e-Biotin-ST-405, PE-anti-CD4 (GK1.5), APC-anti-CD8 (53-6.7) for T cells; Alexa647 anti-B220 (RA3-6B2; eBioscience) for B cells; F4/80-PB for monocytes; and PE-anti-Gr-1 granulocytes (51-01212J; BD Biosciences) (these antibodies were used at 1:100). Cell-cycle analysis BrdU incorporation was analysed with the APC-BrdU Flow Kit (BD Biosciences). BM was assayed 48 h after a single intraperitoneal injection of BrdU (100 μl of a 10 mg ml −1 solution). Surface staining for lineage markers was performed as above with antibodies to Lin-APC-Alexa750, Sca1-Biotin-Qdot605, cKit-PerCP/Cy5.5, CD135-APC and CD34-FITC (GFP is lost after fixing; data not shown). For the apoptosis assay, BM cells were stained with lineage, stem and progenitor markers, followed by staining with DAPI (Molecular Probes) and AnnexinV–APC (BD Biosciences). To detect quiescent HSCs, unmanipulated BM cells were incubated with 10 μg ml −1 Hoechst 33342 for 90 min at 37 °C. Cells were washed and stained with antibodies against cKit, Sca1 and Lin. The cells were fixed in 5% PFA and incubated with the RNA dye Pyronin Y (PY, 1 μg ml −1 ) before flow cytometry. The proportion of cells in G 0 (PY low Hoechst low ) was measured in the LK + S + CD34 low -gated populations. Gene expression and qRT–PCR Total RNA was isolated from PB, BM, spleen and other tissues with the Trizol reagent (Invitrogen), and treated essentially as described [48] , using the primers listed in Supplementary Table S2 . Gene expression analysis is described in Supplementary Information . Chromatin immunoprecipitation assays ChIP was performed essentially as described [48] . Antibodies for immunoprecipitation were rabbit polyclonals to H3K27me3, H3K9me3, H2Aub1, IgM, Ezh2 and H3K4me3 (all from Upstate; 1:2,500). DNA from precipitated complexes was amplified by RT–PCR, performed in triplicate with multiple dilutions, using the primers listed in Supplementary Table S3 . For retroviral transduction of short hairpin RNAs, Ezh2 targeting short interfering RNA (Dharmacon D-00210-01 and D-004218-01) and non-targeting controls were cloned into the pSuper vector (OligoEngine). LSK cells (5×10 5 ) isolated from Ezh2-KI and control mice were infected with shEzh2 or control retrovirus (at least 10 6 cfu ml −1 ) by spinoculation (at 1,600× g and 37°C). After 24 h culture in medium containing 10 ng ml −1 IL-3, 10 ng ml −1 IL-6, and 100 ng ml −1 stem cell factor, a second round of spinoculation was performed, followed by culture for an additional 24 h. Colony assays Lin negative cells (10 4 ) from BM of both genotypes were plated in 1.3%. methylcellulose (H4100, Stem Cell Technologies) supplemented with 30% FBS, 10% detoxified BSA (Stem Cell), 200 mM nonessential amino acids, 200 mM L -glutamine, 10 U ml −1 penicillin G, 10 μg ml −1 streptomycin, 100 M 2-ME (Sigma), 50 μg ml −1 ascorbic acid (Sigma), 20 ng ml −1 IL-6, 20 ng ml −1 mSCF, 10 ng ml −1 mIL-11, 20 ng ml −1 mIL-3, 10 ng ml −1 mTPO, 10 ng ml −1 hG-CSF and 1 U ml −1 hEPO (Amgen). All supplements and media were purchased from Invitrogen and cytokines from R&D Systems, except where indicated. Primitive erythroid colonies were scored after 3–4 days in culture. All other colony types were scored after 7–8 days in culture. To assay formation of granulocyte–macrophage colonies (CFU–GM), nucleated BM cells (1×10 5 ) were plated in triplicate on methylcellulose (MethoCult, Stem Cell) supplemented with granulocyte–macrophage colony stimulating factor (GM–CSF) and IL-3, at the indicated concentrations. Colonies (>30 cells) were scored blindly after 12 days, using an inverted microscope. Protein analysis and immunohistochemistry Immunoblots were performed essentially as described [49] . Mouse Ezh2 was detected with monoclonal antibody AC22 (Cell Signaling), H3K27me3 with rabbit polyclonal antibody (Upstate) and β-actin with monoclonal antibody AC-15 (Sigma). Secondary antibody was HRP-linked anti-mouse IgG (DAKO). Signals were detected by enhanced chemiluminescence (GE Lifesicences). For histopathology, femurs were fixed in formaldehyde, decalcified and paraffin embedded. Spleens were treated similarly, with the omission of decalcification. Sections (4.5 μm) were cut and stained with haematoxylin and eosin (H&E) or processed for IHC. Sections for IHC were staining with antibodies to Ezh2 (AC22; Cell Signaling; 1:1,000), F4-80 (T-2006; BMA Biomedicals; 1:1,000), Mac-1 (ab63317, ABCAM; 1:2,000), CD34 (ab8158; ABCAM; 1:2,000), MPO (A0398; DAKO; 1:1,500) and Ki67 (0003110QD; Master Diagnostica; 1: 500). Samples were then incubated with biotinylated anti-mouse IgG followed by avidin-biotin peroxidase complexes (Vector Lab). Statistical methods All data are expressed as the mean±s.d. The statistical significance of differences was measured by unpaired two-tailed Student's t -test; * P <0.05, or ** P <0.001. Accession codes: The microarray data have been deposited in the Gene Expression Omnibus under accession code GSE28369 . How to cite this article: Herrera-Merchan, A. et al . Ectopic expression of the histone methyltransferase Ezh2 in haematopoietic stem cells causes myeloproliferative disease. Nat. Commun. 3:623 doi: 10.1038/ncomms1623 (2012).